Genome-wide association mapping reveals a rich genetic architecture of complex traits inOryza sativa Asian rice, Oryza sativa is a cultivated, inbreeding species that feeds over half of the world's population. Understanding the genetic basis of diverse physiological, developmental, and morphological traits provides the basis for improving yield, quality and sustainability of rice. Here we show the results of a genome-wide association study based on genotyping 44,100 SNP variants across 413 diverse accessions of O. sativa collected from 82 countries that were systematically phenotyped for 34 traits. Using cross-population-based mapping strategies, we identified dozens of common variants influencing numerous complex traits. Significant heterogeneity was observed in the genetic architecture associated with subpopulation structure and response to environment. This work establishes an open-source translational research platform for genome-wide association studies in rice that directly links molecular variation in genes and metabolic pathways with the germplasm resources needed to accelerate varietal development and crop improvement. Understanding the genetic basis of physiological, developmental and morphological variation in domesticated Asian rice ( Oryza sativa ) is critical for improving the quality, safety, reliability and sustainability of the world's food supply. Human population growth, particularly in developing countries where rice is the main source of caloric intake [1] , coupled with climate change and the intensive water, land and labour requirements of rice cultivation [2] , creates a pressing and continuous global need for new, stress tolerant, resource-use efficient, and highly productive rice varieties. To assist in this endeavour, the scientific community has created a wealth of genomic and plant breeding resources, including high-quality genome sequences [3] , [4] , dense SNP maps [5] , [6] , [7] , extensive germplasm collections [6] , [8] , [9] and public databases of genomic information [5] , [6] , [10] , [11] . Despite the availability of these scientific resources, most of what we know about the genetic architecture of complex traits in rice is based on traditional quantitative trait locus (QTL) linkage mapping using bi-parental populations. While providing valuable insights [12] , the QTL approach is clearly not 'scalable' to investigate the genomic potential and tremendous phenotypic variation of the more than 120,000 accessions available in public germplasm repositories. Genome-wide association study (GWAS) mapping makes it possible to simultaneously screen a very large number of accessions for genetic variation underlying diverse complex traits. An extra advantage of the GWAS design for rice is the homozygous nature of most rice varieties, which makes it possible to employ a 'genotype or sequence once and phenotype many times over' strategy, whereby once the lines are genomically characterized, the genetic data can be reused many times over across different phenotypes and environments. Here we present a genome-wide association study in a global collection of 413 diverse rice ( O. sativa ) varieties from 82 countries using a high-quality custom-designed 44,100 oligonucleotide genotyping array. For these varieties, we systematically phenotyped 34 morphological, developmental and agronomic traits over two consecutive field seasons. Our mapping strategy evaluated variation both within and among four of the major subgroups of rice, revealing significant heterogeneity of genetic architecture among groups, as well as gene-by-environment effects. Unlike previous GWAS studies in rice [5] , purified seed stocks of the rice strains and all the genotypic and phenotypic information generated over the course of this study are publicly available, creating a valuable, open-source translational research platform that can be rapidly expanded through community participation to enhance the power and resolution of GWAS in rice. Diversity panel and genotyping array A rice diversity panel consisting of 413 inbred accessions of O. sativa collected from 82 countries ( Fig. 1 ; Supplementary Data 1 ) was genotyped using an Affymetrix single nucleotide polymorphism (SNP) array containing 44,100 SNPs (hereafter referred to as the 44 K chip). With a genome size of ∼ 380 Mb (ref. 13 ), this custom-designed genotyping chip provides high quality data (less than 4.5% missing data), with ∼ 1 SNP per 10 kb across the 12 chromosomes of rice (Methods; Supplementary Data 2 ). The diversity panel was evaluated for 34 traits related to plant morphology, grain quality, plant development and agronomic performance using field-grown plants with replications within and between years ( Supplementary Table S1 ; Supplementary Data 3 ). 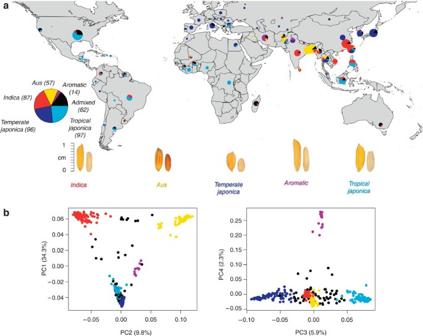Figure 1: Population structure inO. sativa. (a) The large pie chart summarizes the distribution of subpopulations in the 413O. sativasamples in our diversity panel, and the smaller pie charts on the world map correspond to the country-specific distribution of subpopulations sampled (note: large countries such as China, India and the US were divided into several major rice growing regions). The size of the pie chart is proportional to the sample size and colours within each pie chart are reflective of the percentage of samples in each subpopulation. Seeds representing each subpopulation are displayed with and without hull in the centre, with 1 cm scale bar. (b) Principal component analysis was used to provide a statistical summary of the genetic data, and the top four principle components are illustrated in the bottom panels. Figure 1: Population structure in O. sativa . ( a ) The large pie chart summarizes the distribution of subpopulations in the 413 O. sativa samples in our diversity panel, and the smaller pie charts on the world map correspond to the country-specific distribution of subpopulations sampled (note: large countries such as China, India and the US were divided into several major rice growing regions). The size of the pie chart is proportional to the sample size and colours within each pie chart are reflective of the percentage of samples in each subpopulation. Seeds representing each subpopulation are displayed with and without hull in the centre, with 1 cm scale bar. ( b ) Principal component analysis was used to provide a statistical summary of the genetic data, and the top four principle components are illustrated in the bottom panels. Full size image Population structure and linkage disequilibrium estimation in rice Using principle component analysis (PCA) [14] to summarize global genetic variation in the diversity panel, we observed clear, deep subpopulation structure in this collection of germplasm ( Fig. 1a ). The top four principal components (PCs) explained almost half of the genetic variation ( Fig. 1b ). The five subpopulations indica , aus , temperate japonica , tropical japonica and aromatic formed clear clusters based on the top four PCs, and were well differentiated from each other, with pairwise Fst (F-statistic) values ranging from 0.23–0.53. This is in agreement with previous findings where global germplasm collections have been used in combination with much smaller numbers of SNP or simple sequence repeat (SSR) genotypes [8] , [15] , [16] , [17] . Because the array was designed to assay variation in all O. sativa groups, most SNPs are shared or polymorphic across subpopulations ( Table 1 ). Table 1 Polymorphism summary of Affymetrix 44 K SNPs in each subpopulation. Full size table We examined allele sharing across the panel by calculating 'identity by state' coefficients among all pairs of accessions ( Fig. 2a ). We find that whereas allele sharing clearly tracks subpopulation ancestry as identified by the PCA analysis, there is also a substantial number of admixed accessions, highlighting the complex history of rice varieties grown throughout the world [16] . Excluding the small sample of aromatic accessions, the mean observed identical by state (IBS) sharing is greatest between the closely related tropical japonica and temperate japonica accessions (0.80), followed by indica and aus (0.64), with relatively little IBS sharing between the two major subspecies, Indica and Japonica (0.47) ( Fig. 2a ). The fact that most of the admixture occurs within (rather than between) subspecies underscores the existence of genetic and cultural barriers to genetic exchange between these two major groups of Asian rice, despite documented cases of targeted Japonica-Indica introgression mediated by artificial selection [18] , [19] . 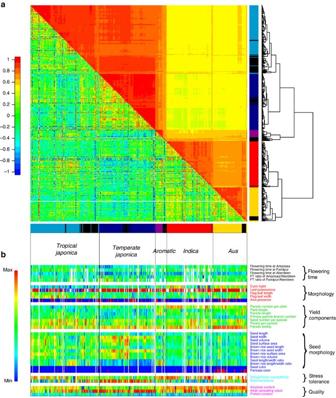Figure 2: Identity by State and phenotypic variation among subpopulations. (a) Individuals are ordered according to their genotypic distance (1-IBS, identified by state) clustering with the tree shown on the right. The upper diagonal shows the IBS-sharing between individuals (values rescaled from 0 to 1). The lower diagonal shows the individual correlation coefficients based on all phenotypes. Coloured bars along the bottom of the panel reflect the sample subpopulation assignment as labelled; dark colour within each subpopulation indicates admixed individuals. (b) Summary of phenotypic distributions among all individuals, with phenotypes grouped by trait category and individuals grouped by subpopulation as in (a). Figure 2: Identity by State and phenotypic variation among subpopulations. ( a ) Individuals are ordered according to their genotypic distance (1-IBS, identified by state) clustering with the tree shown on the right. The upper diagonal shows the IBS-sharing between individuals (values rescaled from 0 to 1). The lower diagonal shows the individual correlation coefficients based on all phenotypes. Coloured bars along the bottom of the panel reflect the sample subpopulation assignment as labelled; dark colour within each subpopulation indicates admixed individuals. ( b ) Summary of phenotypic distributions among all individuals, with phenotypes grouped by trait category and individuals grouped by subpopulation as in ( a ). Full size image The amount of genomic variation tagged by our SNP array was calculated by measuring the pairwise SNP linkage disequilibrium (LD) among the 44 K common SNPs. On average, LD drops to almost background levels around 500 kb–1 Mb, reaching half of its initial value at ∼ 100 kb in indica , 200 kb in aus and temperate japonica , and 300 kb in tropical japonica ( Supplementary Fig. S1 ). Given that our average inter-marker distance is 10 kb, we expect to have reasonable power to identify common variants of large effect associated with our traits of interest, even if we have not queried the causal variant for association in the domesticated varieties. Phenotypic variation The phenotypes we examined in our GWAS can be classified broadly into six categories: plant morphology-related traits; yield-related traits; seed and grain morphology-related traits; stress-related phenotypes; cooking, eating and nutritional-quality-related traits; and plant development, represented by flowering time, which we measured in three geographic locations that differed in day-length and ambient temperature. Canonical correlation analysis demonstrated that phenotypes within a category are often correlated, ranging from a low of −0.41 between brown rice seed width and brown rice seed length, to a high of 0.9 between hulled and dehulled seed morphology ( Fig. 2b ; Supplementary Fig. S2 ). For all the phenotypes evaluated in this study, we observed global similarities among members of the same subpopulation, consistent with the domestication and breeding history of these varieties. Correlation coefficients between accession pairs across all phenotypes were significantly higher for accession pairs from the same subpopulation than from different subpopulations ( P <2.2e−16, one-sided Mann–Whitney U -test) (lower triangle of Fig. 2a ). Consistent with this observation, the top four PCs (based on the 44 K SNPs mentioned above) explained a large proportion of phenotypic variation, with values ranging from 20–40% ( Supplementary Table S1 ). In the case of rice grain, morphological and cooking-quality traits are key to varietal identity and have been under strong diversifying selection by humans in different parts of the world [18] , [19] , [20] , [21] . Physical grain characteristics in rice are salient because they serve as indicators of local and regional eating preferences in a crop that, unlike wheat or maize, is consumed largely as whole kernel. Traits such as flowering time and disease resistance are also strongly correlated with region and environment, meaning that genotypic, phenotypic and environmental variation in O. sativa are all correlated to some degree, posing significant challenges for GWAS. The strong confounding effect of population structure The results of our genome-wide association scans are summarized in Supplementary Figures S3-S36 where we show SNP-trait associations discovered in the diversity panel as a whole, as well as in each subpopulation individually. As can be seen in the quantile–quantile plots ( Fig. 3a ; Supplementary Figs. S3-S36 ), the distribution of observed −log10 P -values from the naïve analysis (no population structure adjustment) departed quite far from the expected distribution under a model of no association (that is, the P -values should lie on the diagonal line), with significant inflation of nominal P -values leading to a high level of false positive signals. Use of a modified mixed model strategy [22] , [23] , [24] allowed us to consider different levels of population structure and relatedness in our diversity panel. This effectively eliminated the excess of low P -values for most traits, but it also likely eliminated true positives. This is a common problem seen in other systems as well; for example, geographic coordinates correlate closely with flowering time in plants [24] . For this reason, we believe a combination of naïve and population structure-adjusted hits, coupled with subpopulation-specific analyses in rice, is the most thoughtful way to identify potential variants for follow up. 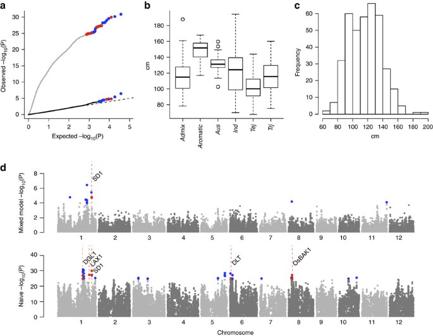Figure 3: Phenotypic distribution and genome-wide association scan for plant height. (a) Quantile–Quantile plots for both naïve and mixed model for plant height in all samples. (b) Boxplot showing the differences in plant height among subpopulations. Box edges represent the upper and lower quantile with median value shown as bold line in the middle of the box. Whiskers represent 1.5 times the quantile of the data. Individuals falling outside the range of the whiskers shown as open dots. (c) Histogram of plant height in all samples. Dashed black line represents the null distribution. (d) Genome-wideP-values from the mixed model and naïve method.xaxis shows the SNPs along each chromosome;yaxis is the −log10(P-value) for the association. Coloured dots in (a) and (c) indicate SNPs withP-values <1×10−4in the mixed model and the top 50 SNPs in the naïve method; SNPs within 200 kb range of known genes are in red; other significant SNPs are in blue. Candidate gene locations shown as red vertical dashed lines with names on top. Figure 3: Phenotypic distribution and genome-wide association scan for plant height. ( a ) Quantile–Quantile plots for both naïve and mixed model for plant height in all samples. ( b ) Boxplot showing the differences in plant height among subpopulations. Box edges represent the upper and lower quantile with median value shown as bold line in the middle of the box. Whiskers represent 1.5 times the quantile of the data. Individuals falling outside the range of the whiskers shown as open dots. ( c ) Histogram of plant height in all samples. Dashed black line represents the null distribution. ( d ) Genome-wide P -values from the mixed model and naïve method. x axis shows the SNPs along each chromosome; y axis is the −log 10 ( P -value) for the association. Coloured dots in ( a ) and ( c ) indicate SNPs with P -values <1×10 −4 in the mixed model and the top 50 SNPs in the naïve method; SNPs within 200 kb range of known genes are in red; other significant SNPs are in blue. Candidate gene locations shown as red vertical dashed lines with names on top. Full size image Using the mixed model [23] to analyse the associations between 34 phenotypes and 44 K SNP genotypes evaluated in our 413 O. sativa rice lines, we successfully identified both known associations (for example, enrichment in a priori candidate genes and previously reported QTLs from rice and other species) as well as new candidate loci in the rice genome. Detailed results for each of the 34 phenotypes can be found in the Supplementary Data 3 as well as online in the Gramene database ( www.gramene.org ) and on our project website ( www.ricediversity.org/44kgwas ). Trade offs between the mixed model and naïve model Plant height is an important developmental and yield-related trait. Dozens of genes regulating plant height in rice have been identified previously including dwarfing mutants [25] , QTLs [12] , orthologues from other plant species, and genomic targets of fine-mapping experiments related to harvest index and yield [12] , [26] . Both the naïve and the mixed model consistently detected strong signal linked to the Green Revolution semi-dwarf gene, SD1 , on chromosome 1 ( Fig. 3d ). Interestingly, several SNPs near other height-controlling genes such as OsBAK1 on chromosome 8 (ref. 27 ), DGL1 on chromosome 1 (ref. 28 ) were only detected by the naïve approach ( Fig. 3d ). This suggests that, in the case of rice, the mixed model may overcompensate for population structure and relatedness, leading to false negatives. Therefore, the many mapping resources derived from crosses between parents belonging to different subpopulations and Oryza species will be needed to complement GWAS, helping to reduce the rate of false positives and false negatives [24] , yielding QTLs that cannot be identified by mapping within subpopulations [29] . Genetic heterogeneity across subpopulations In our diversity panel, aromatic varieties had the longest mean panicles (30 cm), temperate japonica had the shortest (21 cm), aus and indica had intermediate panicle length, and the greatest range of panicle length was observed among tropical japonica varieties ( Fig. 4a ). 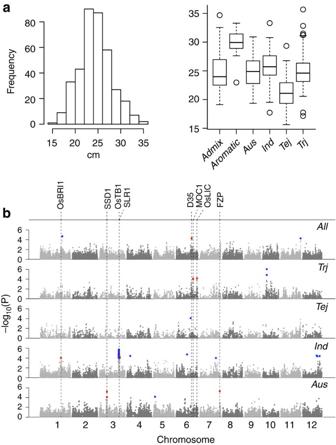Figure 4: Genetic heterogeneity of panicle length across subpopulations. (a) Histogram showing distribution of panicle length across the diversity panel and boxplot showing differences in panicle length among subpopulations. In boxplot, the box edges represent the upper and lower quantile with median value shown as bold line in the middle of the box. Whiskers represent 1.5 times the quantile of the data. Individuals outside of the range of the whiskers shown as open dots. (b) Genome-wideP-values from the mixed model for panicle length for all 413 accessions in top panel (all), and fortropical japonica,temperate japonica,indicaandaussubpopulations individually in subsequent panels. Note: thearomaticsubpopulation was not included because of the small sample size.X-axis indicates the SNP location along the 12 chromosomes;yaxis is the −log10(Pvalue) from each method. Coloured dots indicate SNPs withP-values <1×10−4in the mixed model; SNPs within 200 kb range of known genes are in red; other significant SNPs are in blue. Candidate genes near peak SNP regions known to be previously associated with panicle, stem and internode elongation in rice are shown along the top. Figure 4: Genetic heterogeneity of panicle length across subpopulations. ( a ) Histogram showing distribution of panicle length across the diversity panel and boxplot showing differences in panicle length among subpopulations. In boxplot, the box edges represent the upper and lower quantile with median value shown as bold line in the middle of the box. Whiskers represent 1.5 times the quantile of the data. Individuals outside of the range of the whiskers shown as open dots. ( b ) Genome-wide P -values from the mixed model for panicle length for all 413 accessions in top panel ( all ), and for tropical japonica , temperate japonica , indica and aus subpopulations individually in subsequent panels. Note: the aromatic subpopulation was not included because of the small sample size. X -axis indicates the SNP location along the 12 chromosomes; y axis is the −log 10 ( P value) from each method. Coloured dots indicate SNPs with P -values <1×10 −4 in the mixed model; SNPs within 200 kb range of known genes are in red; other significant SNPs are in blue. Candidate genes near peak SNP regions known to be previously associated with panicle, stem and internode elongation in rice are shown along the top. Full size image To determine whether different networks of alleles were associated with trait variation in the different subpopulations, we performed GWAS on each subpopulation independently and in the panel as a whole, and compared results. As summarized in Figure 4a,b , the genetic architecture of panicle length differs significantly among subpopulations and different GWAS peaks are observed when the subpopulations are analysed individually or when the diversity panel is analysed as a whole. For example, in the indica population, we see clusters of highly significant SNPs near OsTB1 [ TEOSINTE BRANCHED1 (ref. 30 )], SLR1 [ SLENDER RICE1 (ref. 31 )] and OsBRI1 [syn. DWARF61 , or BRASSINOSTEROID-INSENSITIVE1 (ref. 32 )], in the aus subpopulation we observe significant SNPs near FZP [ FRIZZY PANICLE [33] ] and SSD1 [ SWORD SHAPE DWARF1 (ref. 34 )], and in the tropical japonica population, we see SNPs near OsLIC [LEAF AND TILLER ANGLE INCREASED CONTROLLER [35] ] and MOC1 ( MONOCLUM 1 (ref. 36 )). From these results, we conclude that different networks of genes regulate panicle length in different subpopulations and propose that subpopulation-derived genetic heterogeneity is a general pattern in O. sativa . This suggests that the Indica and Japonica varietal groups should be properly treated as true sub-species for association analyses, and helps explain why crosses between members of divergent subpopulations, as well as between cultivated and wild species, often give rise to transgressive offspring [37] . We also demonstrate that the subpopulations of O. sativa contain alleles with vastly different effect-size on many traits of interest (that is, allele effects that are in the opposite direction to mean subpopulation differences for those traits). This conforms to the general mechanism that explains the production of extreme, or transgressive, phenotypes at both the species level and below [37] , [38] and suggests a blueprint for harnessing natural variation to liberate transgressive phenotypes in the context of plant improvement. Genotype by environment effects To investigate how environmental variation affected the performance of GWAS, we evaluated flowering time in three different environments and compared results. One experiment was conducted during 2007 in the field in Stuttgart, Arkansas, USA (34°4′) under long-day conditions ( ∼ 14–12 h during May–September); one was conducted in the field in Faridpur, Bangladesh (23°5′) under ∼ 12–13 h days (January–May); and the third was conducted in the greenhouse in Aberdeen, Scotland, UK (57° 9′) across a nine-month period during which the days became very long and then very short (a range of ∼ 18–6 h during the period spanning March–December). The GWAS peaks explained between 5–50% of the phenotypic variation for flowering time in each environment ( Supplementary Data 4 ). 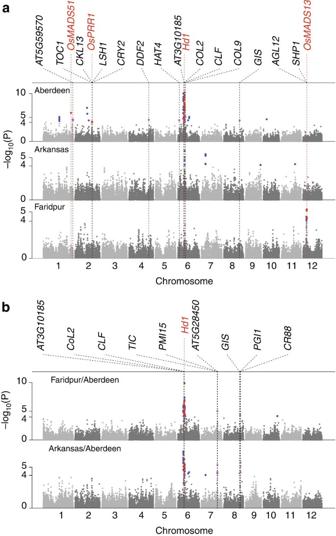Figure 5: Genome-wide association scan for flowering time. (a) Genome-wideP-values from the mixed model for flowering time in three geographic locations are shown in the three panels. Association analysis in each subpopulation is shown in each row of the matrix.Xaxis indicates the SNP location along the 12 chromosomes, with chromosomes separated by vertical grey lines;yaxis is the −log10(Pvalue) from each method. Candidate genes previously shown to determine flowering time near peak SNPs are shown along the top, rice genes are in red,Arabidopsishomologues are in black. SNPs withPvalue <1×10−4are indicated by coloured dots. SNPs within 200 kb range of known rice flowering time genes are in red; SNPs within 200 kb range ofArabidopsisflowering-time homologues are in magenta; other significant SNPs are in blue. (b) GWAS regions associated with photoperiod sensitivity, calculated as the ratio of days-to-flowering across pairs of environments. As seen in Figure 5a , 10 genomic regions were associated with candidate genes for flowering time under one or more daylengths while only the HEADING DATE 1 ( HD1 ) region on chromosome 6 was detected in more than one environment. Figure 5: Genome-wide association scan for flowering time. ( a ) Genome-wide P -values from the mixed model for flowering time in three geographic locations are shown in the three panels. Association analysis in each subpopulation is shown in each row of the matrix. X axis indicates the SNP location along the 12 chromosomes, with chromosomes separated by vertical grey lines; y axis is the −log 10 ( P value) from each method. Candidate genes previously shown to determine flowering time near peak SNPs are shown along the top, rice genes are in red, Arabidopsis homologues are in black. SNPs with P value <1×10 −4 are indicated by coloured dots. SNPs within 200 kb range of known rice flowering time genes are in red; SNPs within 200 kb range of Arabidopsis flowering-time homologues are in magenta; other significant SNPs are in blue. ( b ) GWAS regions associated with photoperiod sensitivity, calculated as the ratio of days-to-flowering across pairs of environments. Full size image The most significant signal was observed under very long days in Aberdeen around HD1 , the major photoperiod-sensitivity locus, (synonym: SE1 , or OsCONSTANS , OsCO ) on chromosome 6 (ref. 39 ). A well-defined peak in the same location was observed under long days in Stuttgart, AR when either the entire diversity panel or the temperate japonica subpopulation was analysed. The significant SNPs detected in Aberdeen covered an extensive region of ∼ 2.3 Mb around HD1 , corresponding to a 'mountain range' as described by Atwell et al . [40] The 'mountain range' distribution may be due to the presence of several linked genes that contribute to flowering time across the region, and/or to the presence of multiple alleles at the HD1 locus, along with multiple introgression events that have been documented within a 5.5 Mb region around the HD1 gene [41] . In domesticated species like rice, loci that are critical to both local adaptation and yield performance are often the targets of both natural and artificial selection, leading to complex forms of allele sharing and admixture in diverse varieties. Some varieties were highly sensitive to daylength and others, mostly temperate japonica accessions, were insensitive to photoperiod and flowered at similar times across the three environments. When photosensitivity (the ratio of days-to-flowering across pairs of environments) was used as a derived trait for GWAS, the most significant SNPs ( P <10 −6 ) were consistently found near HD1 , followed by a region on chromosome 7 containing homologues of Arabidopsis genes known to regulate the circadian rhythm [that is, TIME FOR COFFEE, TIC [42] ] and light sensing [ PLASTIC MOVEMENT IMPAIRED 15 , PMI15 [43] ] ( Fig. 5b ), which have not previously been shown to be associated with natural variation for flowering time in rice. We also demonstrate the effect of genotype by environment (GxE) interaction for flowering time by comparing GWAS results over two years in the same location in Stuttgart, Arkansas ( Supplementary Fig. S37 ). In this case, we observe extensive year-to-year variation between 2006 and 2007, mostly due to the different weather patterns experienced during the two growing seasons. Several GWAS peaks associated with candidate genes are significant in only a single year. The HD1 locus was significant in 2007, but not in 2006, though it was significant using the average flowering time from two years. Although the genetic complexity and low heritability of flowering time as well as several other traits evaluated here in field grown plants ( Supplementary Figs S37-S40 ) tend to confound the interpretation of GWAS results, this study provides an opportunity to look carefully at a range of ecologically and agronomically important traits evaluated under natural growing conditions and compare GWAS results with prior QTL and mutant studies to better understand plant growth and development [44] , [45] . 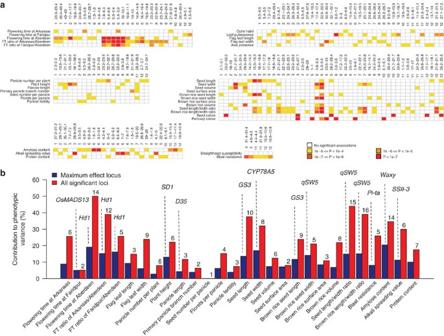Figure 6: Summary of trait associations across genomic regions and percentage of variance explained by significant locus. (a) Each row represents a trait, and each column corresponds to a genomic region containing multiple SNPs that are significantly associated with a trait. Significance is colour-coded based on thePvalue of the association. (b) Thexaxis represents the trait, theyaxis shows the contribution (%) of significant loci. Candidate genes detected within 200 Kb region of significant loci are labelled on top of the maximum effect locus. Gene linkage or pleiotropy A matrix summarizing the QTL regions associated with all traits, as well as the percent of the phenotypic variation explained by significant SNPs for each trait, can be found in Figure 6 . For many traits, the maximum-effect locus falls within a 200 kb region containing a previously identified functional gene (as highlighted in Fig. 6b and summarized in Supplementary Data 4 ). When our results are compared with those of Huang et al . [5] , the same known genes showed clear signal for the same phenotypes (for example, GS3 and qSW5 for grain length and width, SSII-3 and Waxy for alkaline spreading value and amylose content, Rc for pericarp colour). The significant SNPs in our study explained up to 58% of the variance compared with values up to 68% reported by Huang et al . [5] In addition, we evaluated traits not previously documented and identified known genes associated with those traits (for example, SD1 for plant height, OsMADS13 for flowering time and Pi-ta for blast resistance). This demonstrates that our 44 K SNP array is capable of capturing the major common variants responsible for critical agronomic traits. Figure 6: Summary of trait associations across genomic regions and percentage of variance explained by significant locus. ( a ) Each row represents a trait, and each column corresponds to a genomic region containing multiple SNPs that are significantly associated with a trait. Significance is colour-coded based on the P value of the association. ( b ) The x axis represents the trait, the y axis shows the contribution (%) of significant loci. Candidate genes detected within 200 Kb region of significant loci are labelled on top of the maximum effect locus. Full size image In several cases, the same SNPs were significantly associated with multiple traits. This could be the result of pleiotropy or closely linked genes (local LD) [46] . For example, we observed SNPs at 31 Mb chromosome 4 that were significantly associated with both rice blast disease resistance and flag leaf width, and SNPs associated with rice blast disease resistance, amylose content and flowering time at 4.2–4.6 Mb on chromosome 6. These associations were also supported by Canonical correlation analysis based on traits measured in Arkansas ( Supplementary Fig. S2 , r =−0.3 for blast resistance and flag leaf width, r =−0.31 for blast resistance and flowering time, r =0.37 for amylose content and flowering time). Similar trait associations have been previously reported in these and other regions in rice [47] , [48] , [49] . Linkage among favourable alleles is a strong determinant of phenotypic value under both natural and artificial selection, a fact long appreciated by plant breeders. Validation studies involving joint linkage and association mapping, coupled with fine-mapping to identify the exact genes and alleles underlying our GWAS hits, will be required to more clearly understand the relationship between these candidate genes and the phenotypes observed in our panel [46] , as well as to provide breeders with the appropriate genomic tools needed to break deleterious linkages and liberate valuable alleles in this region. The deep population structure of O. sativa and its importance in explaining the heterogeneity of genetic architecture associated with most complex traits in rice underscores the value of using a world-wide diversity panel to untangle the genotype—phenotype associations in the species. As demonstrated by our study, no single GWAS design or analysis method is sufficient to unravel the complex genetics underlying natural variation in O. sativa. The naïve approach has high false positive rates, and, although the mixed model successfully reduces inflation of P -values, it often masks true QTLs that are strongly correlated with population structure. In cases where alleles segregate across multiple subpopulations, the mixed model has the best power to find them. However, when alleles segregate in only one subpopulation, or totally different alleles are present in different subpopulations, the naïve approach detects strong signals in the cloud of other, false signals, while the mixed model approach misses them entirely. As demonstrated by the IBS and Fst estimates, both divergence and heterogeneity among subpopulations is characteristic of the genomic pattern observed in rice. Subdividing the diversity panel to analyse subpopulations independently, using the mixed model, appears to provide a reasonable solution to this problem. Given our marker density and sample size, this study is adequately powered to find alleles of large effect that are common across populations, but a larger panel coupled with higher density of SNPs would empower us to detect more QTLs of small effects. It is noteworthy that some of the strongest signals are quite far from known candidate genes. This may be due, in part, to ascertainment bias where our best tag-SNP for a candidate gene is relatively far from the predicted locus, or we may be tagging previously undiscovered loci that happen to map near a known candidate. SNPs in high LD and with similar allele frequencies would give similar P -values in association. The SNPs used in our study were discovered by array-based re-sequencing of 20 O. sativa accessions across ∼ 100 Mb of the genome [6] . Genetic variation discovered from deep next-generation sequencing in a larger number of accessions is likely to provide improved estimates of LD decay and more highly resolved views of local LD patterns in each subpopulation. Likewise, the integration of transcriptome data will improve our ability to detect moderate strength and rare alleles, as well as to begin to dissect the GxE effects and provide better resolution for the hits found in this study. Recent work by Nicolae [50] suggests that many trait-associated SNPs are likely to be eQTLs, and, in the case of flowering time, there is abundant molecular evidence showing that gene expression levels contribute directly to trait variation [44] . Thus, the trajectory of GWAS in rice is similar to advances in human genetics, where initial studies employed several hundred and then thousands of individuals for common alleles, and subsequent work has been necessary to find associations with either rare alleles or alleles of smaller effect [51] . Our results demonstrate that different traits have different genetic architectures. This reflects the relative strength of environmental and human selection, with corresponding impacts on the phenotypic contribution of maximum effect and the total number of significant SNPs. In some cases, a few genes in a pathway may lead to major changes in adaption, such as HD1 . In other cases, humans may exert selection in different directions on the same gene(s), such as seed length ( GS3 ) [52] amylose content [21] , and aroma [19] . Where domestication-related loci are involved, we often see SNPs with large effect that are shared across different populations [53] , and while they clearly distinguish O. sativa from its wild ancestors, these SNPs of large effect are often difficult to detect in O. sativa , because they are nearly fixed in cultivated material. Other SNPs, even those with only small effects, may be clearly identifiable within individual populations. The subpopulation-specific allele distribution explains why crossing wild and domesticated rice, or one subpopulation with another results in transgressive variation in the progeny [37] . Both linkage drag and pleiotropic effects of a target gene can be either beneficial or troublesome in the context of plant breeding [54] , [55] , and it is helpful to understand the underlying genetic cause of multiple trait associations. In the case of blast resistance, many late-maturing, tropical indica varieties that are resistant to blast disease are used as donors to introduce disease resistance into susceptible, early maturing temperate japonica varieties [16] . However, undesirable traits such as late flowering or inappropriate grain quality, may be co-introduced along with the disease resistance [48] . The use of a broad diversity panel in GWAS not only serves to map associations between traits and DNA polymorphisms but also allows us to unravel the origin of genetic correlations among phenotypic traits, that is, pleiotropy versus genetically linked genes, and facilitates the selection of donors with combinations of traits that are likely to be adaptive and selectively advantageous for breeding in target environments. We note that the rice diversity panel presented here represents an immortalized germplasm resource that is accompanied by both genotypic and phenotypic information ( Supplementary Figs S3-S36 ). The seeds are publicly available through the Genetic Stocks Oryza center in Stuttgart, AR ( http://www.ars.usda.gov/Main/docs.htm?docid=8318 ) or the International Rice Germplasm Collection at International Rice Research Institute in the Philippines ( http://irri.org/our-science/genetic-diversity/get-and/or-submit-seeds ). This enables people around the world to leverage the results of this project as the basis for continued association mapping without incurring any genotyping expense. The purified lines from this study can be used to generate MAGIC or NAM populations [56] to validate GWAS results and to further dissect the complex interaction among genes and environments that underlies quantitative variation in rice. The genotypic dataset and information about the 44 K SNP chip are publicly available ( www.ricediversity.org/44kgwas and www.gramene.org ) and can be used to design more targeted SNP assays for immediate use in variety identification, seed-purity testing, linkage analysis, pedigree confirmation and molecular breeding [57] , [58] . Our work highlights experimental design strategies and challenges involved in finding genes underlying phenotypic variation and is relevant to other species initiating GWAS, especially those with deep population structure. By launching this GWAS platform, we aim to deepen our understanding of natural variation and its phenotypic consequences, and to open the door to more efficient utilization of the enormous wealth of diversity available in rice germplasm repositories around the world. SNP array development and SNP selection We selected 44,100 SNPs from 2 data sources: SNPs from the Oryza SNP project, an oligomer array-based re-sequencing effort using Perlegen Sciences technology [6] and BAC clone Sanger sequencing of wild species from OMAP project [59] . Priority was given to SNPs with the least amount of missing data across the 20 SNP discovery accessions in the Oryza SNP project. SNPs were selected to tag all 159,879 high quality SNPs in the Oryza SNP data (Intersection set) with criteria of r 2 =1 and a conservative tagging window size of 50 kb. To further filter the SNPs, Blast was performed using the 33 bp sequence flanking each SNP to remove any SNPs that mapped to more than 1 location in the genome with fewer than 2 mismatches. Also, SNP targets were removed if there were SNPs detected within 15 bp of the target in the low-quality Union set (359,000 SNPs) in the Oryza SNP dataset. This yielded 31,663 tagging SNPs. We then selected 8,437 SNPs from a pool of SNPs from the Intersection and Union sets of the Oryza SNP data and another 4,000 SNPs from the OMAP dataset to fill in any gaps >20 Kb between the tagging SNPs. This generated a well-distributed SNP array providing ∼ 1 SNP every 10 kb along the 12 chromosomes of rice. The microarray data has been deposited in the NCBI dbSNP Database under the accession codes 469281739 to 469324700. Target probe preparation and 44 K SNP array hybridization Rice genomic DNA was extracted from young green leaf tissue following Qiagen plant DNeasy protocol. The probe was generated using the BioPrime DNA labeling kit (Invitrogen, Cat. No: 18094-011), and hybridization conditions were based on the Affymetrix SNP 6.0 protocol. Approximately 750 μg to 1 μg of rice genomic DNA was labelled overnight at 25 °C using 3 vol of the BioPrime DNA labelling reactions. The labelled DNA was ethanol precipitated, resuspended in 40 μl H 2 O, and then added to the Affymetrix SNP 6.0 hybridization cocktail. We did not include Human Cot-1 DNA because of the small size of the rice genome and the fact that it has a much smaller proportion of repetitive DNA compared with human or other mammals for which the assay was originally optimized. SNP genotype calling Genotypes are called using our program ALCHEMY, which was designed to provide improved performance in small sample sizes and for inbred populations with very low levels of heterozygosity [60] . SNPs with low quality (that is, low call rate and allele frequency) across all samples were removed from the dataset and 36,901 high-performing SNPs (call rate >70%, minor allele frequency >0.01) were used for all analyses. Of these SNPs, inbred samples had a median call rate of 95.9% and pairwise concordances between technical replicates yielded >99% average pairwise concordance and >92% average call rate. Plant materials The Rice Diversity Panel consists of 413 Asian rice ( O. sativa ) cultivars, including many landraces, which originated from 82 countries, representing all the major rice-growing regions of the world [15] . The panel contains 87 indica , 57 aus , 96 temperate japonica , 97 tropical japonica , 14 groupV/aromatic , and 62 highly admixed accessions. All accessions were purified for two generations (single seed descent) before DNA extraction. In all, 20 of these 413 accessions were purified as part of the Oryza SNP project [6] . Six cultivars (Azucena, Moroberekan, Nipponbare, Dom-Sofid, IR64, M-202) were purified separately, once by Ali et al . [15] and once as part of the Oryza SNP panel. Further information for each accession (accession name, accession number, country of origin and subpopulation ancestry based on PCA) is given in Supplementary Data 1 . Phenotypic evaluation and correlation among individuals Rice accessions were evaluated in the field at Stuttgart, Arkansas during the growing season (May–October) in 2006 and 2007. Two replications per year were grown in a randomized complete block design in single-row plots of 5 m length with a spacing of 25 cm between the plants and 0.50 m between the rows. A brief description of each trait, its acronym, and evaluation methodology are summarized in Supplementary Table S1 . Phenotypic correlations between individuals were calculated based on all phenotypes used in our study. Estimation of LD decay in rice The amount of genomic variation tagged by our SNP array was calculated by measuring the pairwise SNP linkage disequilibrium (LD) among the 44 K common SNPs (with MAF>0.05) using r 2 , the correlation in frequency among pairs of alleles across a pair of markers. For all pairs of autosomal SNPs, r 2 was calculated using the --r2 --ld-window 99999 --ld-window-r2 0 command in PLINK [61] . Of the more than 44,100 SNP variants we assayed, we found 34,454 ( ∼ 78%) with minor allele frequency >0.05 across the O. sativa panel. When calculated across the entire O. sativa panel, LD is small at short distances ( r 2 <0.45 at 5 kb) but then decays more slowly, and still shows substantial residual LD at a distance of 2 Mb, reflecting the deep subpopulation structure ( Supplementary Fig. S2 ). Within each subpopulation, we calculated r 2 between all pairs of SNPs where both SNPs had <20% missing data and MAF≥5%. Population structure Principal component analysis was done using EIGENSOFT [14] . PC1 separates the samples into two main subspecies- Indica and Japonica and explains 34% of the genetic variance whereas PC2 separates indica from aus and explains 10% of the variance. We find that PC3 separates the two japonica groups into temperate and tropical components ( ∼ 6% of the variance), and PC4 identifies the aromatic group as a clear and distinct gene pool ( ∼ 2% of the variance). (1- IBS) values were used as the distance between individuals to construct the hierarchical clustering tree using complete linkage method in Figure 2a . Genome-wide association Association analyses were performed with and without correcting for population structure. A mixed model approach implemented in EMMA [22] was used to correct the confounding of population structure. The relatedness matrix, measured as the genetic similarity between individuals and IBS values (that is, proportion of times a given pair of accessions had the same genotype across all SNPs), was used to estimate random effects. For all samples, SNPs and the top four PCs were used as fixed effects; for association analysis within each subpopulation, only SNPs were used as fixed effects in the model. For analyses without confounding, simple linear regression or logistic regression was used for continuous and binary traits, respectively. All statistical model details are described in the Supplementary Method . Unless explicitly mentioned, when two-year data were available, mean values across replicates and years of phenotypes were used in association analysis throughout the paper. To examine the effect of 'year' on GWAS results, we introduced 'year' as a covariate in the mixed model, along with the SNPs and 4 PCs. We graphed the correlation between P -values using the two-year-phenotypic mean and using 'year' as a cofactor in the model for flowering time and flag leaf length ( Supplementary Fig. S41 ). When examining GxE effects across locations, only 2007 flowering time data from Arkansas was used for consistency with single-year data from the other locations. Candidate genes near hits were extracted from the literature. Rice homologues of Arabidopsis flowering time genes were extracted from the Gramene Database ( www.gramene.org ). Phenotypic variance contribution of significant loci To obtain significant loci from EMMA for each phenotype, all significant SNPs within 200 Kb were consolidated into one lowest P -value SNP to remove linkage disequilibrium. Large LD regions such as Hd1 were also consolidated into one single, most significant SNP. Only continuous traits were considered for variance contribution estimation. SNP contribution to the phenotypic variance was estimated using ANOVA with the R package; statistical model details are provided in the Supplementary Method . Accession codes: The microarray data has been deposited in the NCBI dbSNP Database under the accession codes 469281739 to 469324700. How to cite this article: Zhao, K. et al . Genome-wide association mapping reveals a rich genetic architecture of complex traits in Oryza sativa . Nat. Commun. 2:467 doi: 10.1038/ncomms1467 (2011).